Orthogonal switching of a single supramolecular complex Orthogonal control over systems represents an advantage over mono-functional switches as both the nature and order of distinctly different stimuli manifest themselves in a wide array of outcomes. Host–guest complexes with multiple, simultaneously bound guests offer unique opportunities to address a set of ‘on’ and ‘off’ states accessible on demand. Here we report cucurbit[8]uril-mediated host–guest heteroternary complexes constructed with both redox- and light-responsive guests in a single, supramolecular entity. The complex responds to orthogonal stimuli in a controlled, reversible manner generating a multifunctional switch between a ‘closed’ heteroternary complex, a redox-driven ‘closed’ homoternary complex and a photo-driven ‘open’ uncomplexed state. We exploit both photochemical and electrochemical control over the supramolecular coding system and its surface wettability to demonstrate the system’s complexity, which could be readily visualized on a macroscopic level, thus offering new opportunities in the construction of memory devices. Harnessing external control over a system in an aqueous environment and tuning its properties reversibly on demand has attracted considerable interest across the chemical and biological sciences [1] , [2] , [3] , [4] . The highly dynamic nature of supramolecular non-covalent processes offers versatile tools to utilize and amplify external stimuli in the manipulation of material properties through reversible stimuli-responsive molecular switching [5] . Recent efforts have been dedicated to gaining orthogonal control over supramolecular systems, whereby different responses can be triggered on demand with a specific order of input stimuli, representing versatility and complexity beyond unifunctional systems [6] . One attractive way to achieve this is to delicately combine host–guest molecular recognition with other non-covalent interactions, for example, metal–ligand or protein–ligand interactions [7] , [8] , [9] , [10] . A major limitation in the field, however, has been the incorporation of multiple responsive components into one single supramolecular entity directly. This would serve to overcome any incompatibility between two different types of non-covalent interactions, as well as increase the overall complexity of the system. Among supramolecular stimuli-responsive systems, photosensitive host–guest complexes are of significant interest as light can be applied in a remote manner as an external stimulus and offers precise control over wavelength [11] . In particular, azobenzene derivatives have been extensively used as guests to form inclusion complexes with asymmetric macrocyclic hosts achieving binary photochemical devices [12] , [13] , [14] , [15] , [16] , [17] , based on its well-documented photoisomerism [18] . Although symmetric macrocyclic hosts such as cucurbit[n]urils, ( n =7 and 8) have been used to form either binary inclusion complexes with CB[7] [19] , [20] , or ternary complexes with CB[8] and methylviologen (MV 2+ ) [21] , no photoresponsive CB systems have been demonstrated. Although guests such as stilbene analogues [22] , naphthalene/anthracene derivatives [23] , [24] and coumarins [25] have been used to form 2:1 homoternary complexes with CB[8], their irreversible photodimerizations limit further application in orthogonal switching. As an alternative to photoresponsive systems, redox-responsive host–guest complexes represent another route for constructing supramolecular electromechanical devices [26] , [27] , [28] . Both ferrocene [29] and viologen derivatives [30] , [31] have been used as guests for supramolecular macrocyclic hosts [32] , [33] , [34] , [35] , [36] , [37] . In comparison with ferrocene derivatives, whose sizes only allow for the formation of 1:1 inclusion complexes with such hosts [38] , viologen derivatives have been widely used as guests in ternary complexes with CB[8] [39] , [40] , [41] . Although a variety of applications such as glucose sensing, peptide separation and self-assembly of dendrimers have been reported [42] , [43] , [44] , no previous report has demonstrated an orthogonal response with such a ternary system. Herein, we report the design and construction of orthogonal stimuli-responsive single supramolecular entities based upon CB[8]-mediated heteroternary complexation with viologen and azobenzene derivatives as functional guests in water ( Fig. 1 ). As functionalization of the CB[8] macrocycle is not required for heteroternary complexation, the straightforward self-assembly process represents a versatile platform for the construction of orthogonal stimuli-responsive supramolecular systems. As both molecular guests experience distinct equilibria with the CB[8] host, reversible and orthogonal responses to discrete external stimuli were realised through both light-induced isomerization of azobenzene and redox-driven dimerization of viologen. Furthermore, by surface modification, we demonstrate the amplification of orthogonal stimuli that can be readily visualized on a macroscopic level, and the potential to construct molecular devices with higher complexity. 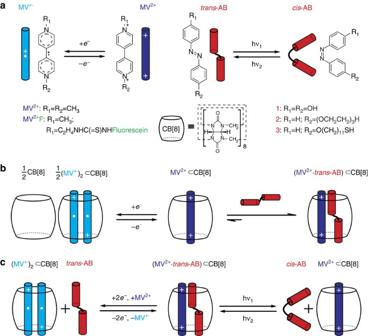Figure 1: Schematic illustration of the design, formation and orthogonal switching of a heteroternary complex. (a) Redox-induced reversible transition between MV2+and MV+·, and light-driven photoisomerization of azobenzene derivatives. (b) Stepwise formation of Cucurbit[8]uril (CB[8])-mediated heteroternary complex with MV2+as the first guest and an azobenzene derivative as the second guest, as well as the one-electron reduction of MV2+CB[8]. (c) The redox-driven reversible transition between a ‘close’ heteroternary complex and a ‘close’ homoternary complex with thetransisomer, as well as the light-driven reversible transition between a ‘close’ heteroternary complex and an ‘open’ inclusion complex with thecisisomer. Figure 1: Schematic illustration of the design, formation and orthogonal switching of a heteroternary complex. ( a ) Redox-induced reversible transition between MV 2+ and MV +· , and light-driven photoisomerization of azobenzene derivatives. ( b ) Stepwise formation of Cucurbit[8]uril (CB[8])-mediated heteroternary complex with MV 2+ as the first guest and an azobenzene derivative as the second guest, as well as the one-electron reduction of MV 2+ CB[8]. ( c ) The redox-driven reversible transition between a ‘close’ heteroternary complex and a ‘close’ homoternary complex with the trans isomer, as well as the light-driven reversible transition between a ‘close’ heteroternary complex and an ‘open’ inclusion complex with the cis isomer. Full size image High selectivity of MV 2+ CB[8] towards trans -azobenzene To investigate the second binding event, a UV/visible (vis) titration was performed between an azobenzene derivative 1 and the preformed complex MV 2+ CB[8]. The relative decrease in absorbance of 1 ( Fig. 2a , 320–500 nm) with a concomitant increase at 251 nm from MV 2+ CB[8] generated an isosbestic point at 317 nm, suggesting the heteroternary complex was indeed formed [20] . The significant quenching of the n-π * absorbance of 1 around 440 nm compared with the slight decrease of the π-π * absorbance at 363 nm suggests the relative abundance of trans - 1 over its cis isomer counterpart upon the heteroternary complexation. One likely explanation is that cis - 1 is geometrically unfavourable to be bound inside the cavity of CB[8] in the presence of MV 2+ ( Supplementary Fig. S1 ) [21] . Another possibility is that the higher polarity of cis - 1 makes it more likely to remain solvated in an aqueous environment rather than be inside the hydrophobic cavity of CB[8]. In contrast, when an aqueous solution of 1 was treated with CB[8], a dramatic colour change was observed from a yellow ( λ max =353 nm) to a dark-red ( λ max =502 nm) solution ( Supplementary Fig. S2a ). This unique colour change indicated the formation of an inclusion complex cis - 1 CB[8], which was confirmed by NMR ( Supplementary Fig. S2b , isothermal titration calorimetry (ITC) was used to determine the binding constant of cis - 1 towards CB[8], but it falls below the lower limit (10 3 M −1 ) of the measurement range) [20] . It is clear from Fig. 2a that no specific cis - 1 -CB[8] interactions occurred in the heteroternary complex as no absorbance was observed at 502 nm. Further confirmation was achieved by a displacement experiment whereby adding MV 2+ into the preformed cis - 1 CB[8] displayed a disappearance of the characteristic colour of cis - 1 CB[8] as a consequence of breaking apart the cis - 1 CB[8] owing to the apparent difference of binding constants (10 5 –10 6 for MV 2+ , thus at least two orders of magnitude higher than that of cis - 1 towards CB[8]). The obvious colour difference between cis - 1 CB[8] (dark red) and (MV 2+ · trans - 1 ) CB[8] (faint yellow) clearly suggested a different selectivity for MV 2+ CB[8] and CB[8] alone as supramolecular hosts for different isomers of 1 . Collectively the data suggest that MV 2+ CB[8] selectively recognized the trans isomer as the better second guest over the cis isomer, leading to the formation of a 1:1:1 heteroternary complex (MV 2+ · trans - 1 ) CB[8]. 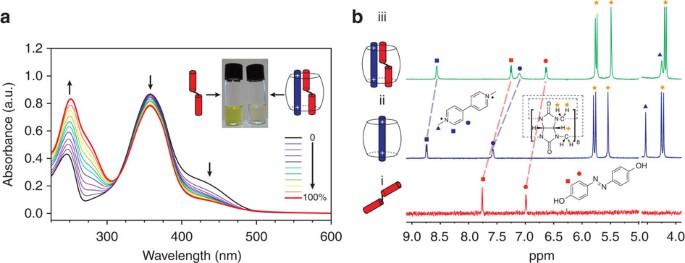Figure 2: Formation of heteroternary complex. (a) UV/vis titration of1upon increasing amount of MV2+CB[8] (molar ratio from 0 to 100%) in water at pH=7 at 25 °C. A 0.05 mM solution of1was kept in dark at 25 °C overnight before starting the titration. Inset: solutions of1at 0.05 mM in water at pH=7 at 25 °C (left) alone, (right) in the presence of an equimolar preformed 1:1 complex MV2+CB[8] (0.05 mM). (b)1H NMR spectra of (i)1, (ii) preformed complex MV2+CB[8] and (iii) heteroternary complex (MV2+·trans-1)CB[8] at 0.5 mM in D2O at pH=7 at 25 °C. The area around HOD peak between 4.6–5.0 ppm was removed for clarity. Figure 2: Formation of heteroternary complex. ( a ) UV/vis titration of 1 upon increasing amount of MV 2+ CB[8] (molar ratio from 0 to 100%) in water at pH=7 at 25 °C. A 0.05 mM solution of 1 was kept in dark at 25 °C overnight before starting the titration. Inset: solutions of 1 at 0.05 mM in water at pH=7 at 25 °C (left) alone, (right) in the presence of an equimolar preformed 1:1 complex MV 2+ CB[8] (0.05 mM). ( b ) 1 H NMR spectra of (i) 1 , (ii) preformed complex MV 2+ CB[8] and (iii) heteroternary complex (MV 2+ · trans - 1 ) CB[8] at 0.5 mM in D 2 O at pH=7 at 25 °C. The area around HOD peak between 4.6–5.0 ppm was removed for clarity. Full size image Formation of (MV 2+ · trans - 1 ) CB[8] was further confirmed by both 1 H NMR spectroscopy and ESI-MS. Significant upfield shifts ( Fig. 2biii ) in the proton spectra of the aromatic region of both 1 and MV 2+ CB[8] were observed compared to those of free 1 ( Fig. 2bi ) and MV 2+ CB[8] ( Fig. 2bii ). This was likely on account of the shielding effect of the CB[8] cavity upon heteroternary complexation in D 2 O. The NMR result was in good accordance with the mass spectrum, which showed a peak at m / z =865.04 corresponding to a doubly charged heteroternary complex [M] 2+ ( Supplementary Fig. S3 ). Photochemical switching upon light-driven isomerization As 1 displayed relatively poor water solubility, it was decided to employ an asymmetric triethylene glycol modified azobenzene derivative 2 to facilitate ITC studies and thus gain a quantitative understanding of the difference in the binding affinity of MV 2+ CB[8] towards the different isomers of azobenzene. As shown in Fig. 3a , when an aqueous solution of MV 2+ CB[8] was titrated with trans - 2 , an isotherm was obtained suggesting a binding constant of 1.44±0.284 × 10 4 M −1 (pH=7 at 25 °C). In comparison, the binding constant between an immediately formed cis - 2 (irradiated under UV light for 20 min) and MV 2+ CB[8] was too weak to be measured by ITC. The combined UV/vis, NMR and ITC data all point to a substantially higher MV 2+ CB[8] selectivity for the trans isomer over the cis isomer upon heteroternary complexation. 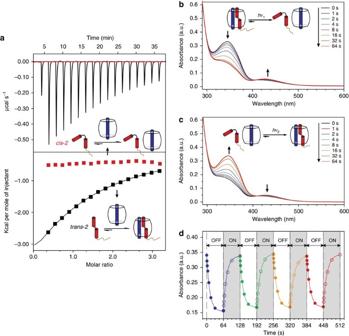Figure 3: Photochemical response of heteroternary complex. (a) Calorimetric titration plots of MV2+CB[8] withcis-2(top, in red) andtrans-2(bottom, in black) in water at pH=7 at 25 °C. ΔG=−23.31 kJ mol−1, ΔH=−19.60±4.69 kJ mol−1, ΔS=−18.79 J K−1mol−1. (b,c) Time-dependent UV/vis spectra of (MV2+·2)CB[8] in water (0.1 mM) under UV light (350 nm) irradiation for 64 s followed by visible light (420 nm) irradiation for 64 s. (d) Kinetic plots of photoresponse of (MV2+·2)CB[8] (λmax=346 nm) during UV and visible irradiation for four cycles. Figure 3: Photochemical response of heteroternary complex. ( a ) Calorimetric titration plots of MV 2+ CB[8] with cis - 2 (top, in red) and trans - 2 (bottom, in black) in water at pH=7 at 25 °C. Δ G =−23.31 kJ mol −1 , Δ H =−19.60±4.69 kJ mol −1 , Δ S =−18.79 J K −1 mol −1 . ( b , c ) Time-dependent UV/vis spectra of (MV 2+ · 2 ) CB[8] in water (0.1 mM) under UV light (350 nm) irradiation for 64 s followed by visible light (420 nm) irradiation for 64 s. ( d ) Kinetic plots of photoresponse of (MV 2+ · 2 ) CB[8] ( λ max =346 nm) during UV and visible irradiation for four cycles. Full size image In the absence of MV 2+ CB[8], 2 exhibited a typical trans–cis isomerization under UV (350 nm) light irradiation, showing a gradual decrease at 343 nm and a concomitant increase at 430 nm, with isosbestic points at both 297 and 419 nm ( Supplementary Fig. S4 ), indicating an equilibrium between the trans and cis isomers. A photo-stationary state was reached after ca. 32 s in water at pH=7 at 25 °C. The decreased absorbance at 343 nm fits a first-order decay and yielded a trans–cis isomerization (confirmed by both 1D and 2D NMR spectra, Supplementary Fig. S5 ) rate constant of 0.296 s −1 . The complementary cis–trans isomerization was achieved by visible light (420 nm) irradiation, with a cis–trans isomerization rate constant of 0.141 s −1 . As expected, upon UV irradiation, (MV 2+ · 2 ) CB[8] (heteroternary complexation was confirmed by both UV/vis and NMR spectroscopy, Supplementary Fig. S6 ) also showed a gradual decrease at 346 nm and a slight increase at 425 nm ( Fig. 3b ), with an isosbestic point at 411 nm, indicating that the heteroternary complex is indeed photoresponsive. The reverse process was readily achieved by visible light irradiation ( Fig. 3c ), and many cycles of alternating UV/visible irradiation could be carried out without any obvious decay ( Fig. 3d ). The apparent isomerization rate constant of 2 in the presence of MV 2+ CB[8] was measured to be 0.080 s −1 , which is 3.7 times slower than that of the trans–cis isomerization of 2 in the absence of MV 2+ CB[8]. This decreased rate constant suggests that heteroternary complexation has a profound effect on the trans to cis isomerization of 2 . As neither MV 2+ or MV 2+ CB[8] absorbs light above 325 nm ( Supplementary Fig. S7 ), the overall isomerization rate of trans - 2 likely depends on the equilibrium between ‘free’ and ‘bound’ 2 in the heteroternary complex. As the k out for 2 is 4 orders of magnitude slower than k in (as measured by ITC in the form of a binding constant), it is therefore reasonable to suggest that trans - 2 undergoes isomerization almost immediately after leaving the CB[8] cavity, thereby ‘locking’ itself out of the CB[8] cavity. Subsequently, upon 420 nm irradiation of the solution, cis to trans isomerization of 2 led to reformation of the heteroternary complex. Together with the binding affinity studies shown in Fig. 3a , the photoirradiation generated a fully reversible transition between an original ‘closed’ heteroternary complex and a dissociated ‘open’ state of MV 2+ CB[8] and cis - 2 . Electrochemical switching upon redox-driven dimerization Methyl viologen exhibits two consecutive one-electron reductions, and was used as the first guest in forming the heteroternary complex on account of its remarkable electrochemical responsiveness. The redox chemistry of viologen in the presence of CB[8] without [45] or with [46] a second guest has been well characterized. As the transition from MV 2+ to MV +· ( Fig. 1a left) drives the formation of the 2:1 homoternary complex (MV +· ) 2 CB[8] ( Fig. 1b left), only the first one-electron reduction of MV 2+ was carried out for the demonstration of the electrochemical response of the heteroternary complex. As shown in Fig. 4ai-ii , the positive shift of ~117 mV observed in the half-wave potential (Δ E 1 p ) of the first one-electron reduction of MV 2+ in the presence of CB[8] is on account of the formation of the homoternary complex (MV +· ) 2 CB[8] [45] . Heteroternary complexation upon addition of second guest 2 induced a smaller positive shift of E 1 p ~87 mV as compared with that of MV 2+ CB[8] ( Fig. 4ai–iii ), showing that the heteroternary complex is indeed electrochemically active. 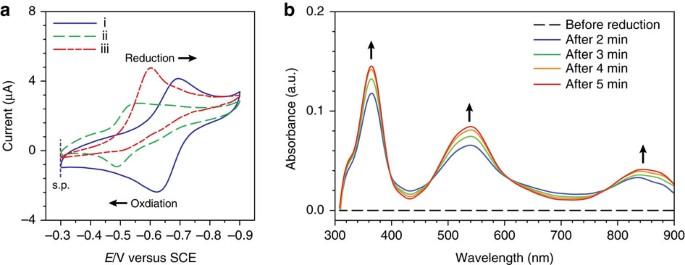Figure 4: Electrochemical response of the heteroternary complex. (a) Cyclic voltammograms of (i) MV2+, (ii) binary complex MV2+CB[8] and (iii) heteroternary complex (MV2+·2)CB[8] (scan rate 0.025 V s−1). Each sample was run at 0.25 mM in 0.1 M phosphate buffer at pH=7; a glassy carbon electrode was used as the working electrode and SCE as the reference electrode (scans start from −0.3 V as indicated by the vertical dashed line in purple, to −0.9 V). (b) UV/vis spectra of (MV2+·2)CB[8] under electrochemical reduction (0.1 mM in 0.25 M phosphate buffer at pH=7) using an indium tin oxide glass electrode as the working electrode (applied potential, −0.7 V versus SCE). SCE, saturated calomel electrode. Figure 4: Electrochemical response of the heteroternary complex. ( a ) Cyclic voltammograms of (i) MV 2+ , (ii) binary complex MV 2+ CB[8] and (iii) heteroternary complex (MV 2+ · 2 ) CB[8] (scan rate 0.025 V s −1 ). Each sample was run at 0.25 mM in 0.1 M phosphate buffer at pH=7; a glassy carbon electrode was used as the working electrode and SCE as the reference electrode (scans start from −0.3 V as indicated by the vertical dashed line in purple, to −0.9 V). ( b ) UV/vis spectra of (MV 2+ · 2 ) CB[8] under electrochemical reduction (0.1 mM in 0.25 M phosphate buffer at pH=7) using an indium tin oxide glass electrode as the working electrode (applied potential, −0.7 V versus SCE). SCE, saturated calomel electrode. Full size image Upon electrochemical reduction at −0.7 V, the formation of (MV +· ) 2 CB[8] was observed by the characteristic absorbance bands centred at 366, 544 and 860 nm ( Fig. 4b ) [45] , confirming the dissociation of (MV 2+ · 2 ) CB[8]. The electrochemical reoxidation of the resulting (MV +· ) 2 CB[8] complex in the presence of 2 regenerated the original heteroternary complex (MV 2+ · 2 ) CB[8], as the characteristic absorbance of (MV +· ) 2 CB[8] completely disappeared and the original absorbance of the heteroternary complex fully recovered ( Supplementary Fig. S8 ). The combined CV and spectroelectrochemical experiments confirmed the redox-driven fully reversible transition between a ‘closed’ heteroternary complex and a ‘closed’ homoternary complex with ‘unbound’ second guest 2 . In an effort to demonstrate that the external stimuli described above are able to act orthogonally in a single supramolecular system, the electrochemical response of the heteroternary complex was investigated under photoirradiation conditions. When (MV 2+ · trans - 2 ) CB[8] was irradiated with UV light (350 nm), a new reduction potential was observed on account of the formation of the dissociation of heteroternary complex. Subsequent visible light (420 nm) irradiation promoted full recovery of the heteroternary complex as an almost identical E pc was observed again in its native peak position, corresponding to that of the original heteroternary complex ( Supplementary Fig. S9 ). A same similar shift trend of the E pa during photoisomerization was also observed, first shifting to that of (MV +· ) 2 CB[8] upon UV irradiation followed by moving back to the original potential ( Supplementary Fig. S9 for scan rate effect on the absolute value of shift). This reversible behaviour clearly indicated that photoirradiation was fully compatible with the redox-responsive nature of MV 2+ CB[8] complexes, and thus offers an orthogonal handle over the supramolecular system. Orthogonal switching on surfaces To demonstrate how this unique orthogonally controlled system can be exploited to amplify different external stimuli, such as light and redox potential into macroscopic properties, the tuning of surface wettability was investigated. To complement previous work, in which a viologen functionalized thiol was used to form a self-assembled monolayer (SAM) on a Au substrate [43] , [47] , a SAM of thiol-containing azobenzene derivative 3 on a Au substrate was prepared by micro contact printing to offer additional characterization of surface wettability ( Supplementary Fig. S10 for the photo-switchability of 3 ). After a 3 -terminated Au substrate was introduced into a solution of preformed (MV 2+ F) CB[8] complex, a 2D fluorescent pattern ( Fig. 5b middle: (1,1) state) was readily visualized on account of the formation of the heteroternary complex (MV 2+ F· 3 ) CB[8]. A 25° decrease in the water contact angle from θ =93° ( Supplementary Fig. S11 ) to θ =68° ( Fig. 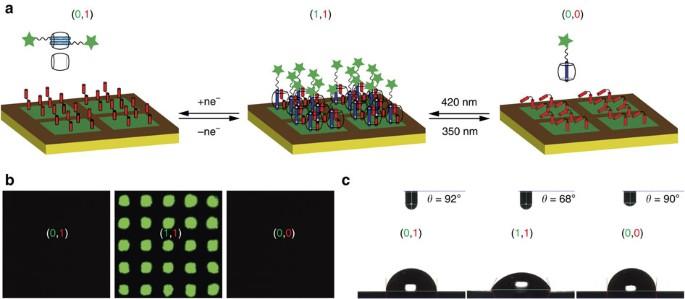Figure 5: Orthogonal switching of the heteroternary complexes on a surface. (a) Schematic illustration of isomerization-driven photoswitching (1,1)↔(0,0) and dimerization-driven electrochemical switching (1,1)↔(0,1). Micro-patterned fluorescent arrays were prepared by the addition of MV2+FCB[8] (5 μM) to the3-terminated Au substrate for 5 min. For photoswitching, the resulting substrate was irradiated by UV light (350 nm) for 1 min in the presence of MV2+FCB[8] followed by visible light irradiation (420 nm, 2 min). For redox switching, the substrate was used as the working electrode for the electrochemical reduction (applied potential: −0.7 V versus SCE) in the presence of 0.1 mM MV2+FCB[8] in 0.1 M phosphate buffer (pH=7) for 5 min followed by electrochemical reoxidation (−0.3 V versus SCE) for 10 min. (b) Fluorescence microscopy images (λex=488 nm) of (left): (0,1) after electrochemical reduction; (middle): (1,1) state with 50 (square dimension) × 50 (interval length) μm arrays (as prepared, after visible light irradiation, and after electrochemical oxdiation); (right): (0,0) state after UV light irradiation. (c) Water contact angle measurement of the corresponding states. 5c middle (1,1)) occurs on account of the presence of positive charges from MV 2+ F. Figure 5: Orthogonal switching of the heteroternary complexes on a surface. ( a ) Schematic illustration of isomerization-driven photoswitching (1,1)↔(0,0) and dimerization-driven electrochemical switching (1,1)↔(0,1). Micro-patterned fluorescent arrays were prepared by the addition of MV 2+ F CB[8] (5 μM) to the 3 -terminated Au substrate for 5 min. For photoswitching, the resulting substrate was irradiated by UV light (350 nm) for 1 min in the presence of MV 2+ F CB[8] followed by visible light irradiation (420 nm, 2 min). For redox switching, the substrate was used as the working electrode for the electrochemical reduction (applied potential: −0.7 V versus SCE) in the presence of 0.1 mM MV 2+ F CB[8] in 0.1 M phosphate buffer (pH=7) for 5 min followed by electrochemical reoxidation (−0.3 V versus SCE) for 10 min. ( b ) Fluorescence microscopy images ( λ ex =488 nm) of (left): (0,1) after electrochemical reduction; (middle): (1,1) state with 50 (square dimension) × 50 (interval length) μm arrays (as prepared, after visible light irradiation, and after electrochemical oxdiation); (right): (0,0) state after UV light irradiation. ( c ) Water contact angle measurement of the corresponding states. Full size image UV light (350 nm, 1 min) irradiation of the resulting substrate in the presence of (MV 2+ F) CB[8] led to the disappearance of the fluorescent array ( Fig. 5b right: (0,0)) and the hydrophobicity of the resulting surface recovered ( θ =90°, Fig. 5c right). This was apparently driven by the photoisomerization of azobenzene (1→0 transition), resulting in the dissociation of (MV 2+ F· 3 ) CB[8]-terminated substrate into a cis - 3 -terminated substrate 0 state, and released (MV 2+ F) CB[8] complex (represented by 0 on account of its absence on surface). The fluorescent pattern could be rewritten onto the surface ((0,0)→(1,1) transition) with a concomitant increase in the surface hydrophilicity ( θ =68°) after irradiating the resulting cis - 3 -terminated substrate with visible light (420 nm, 2 min) in the same MV 2+ F CB[8] solution. It should be pointed out that the cis - 3 -terminated substrate was obtained in the presence of MV 2+ F CB[8] as a fully ‘closed’ state 0 in terms of recognizing other first-guest CB[8] complex unless the cis–trans photoisomerization 0→1 was carried out. A control experiment demonstrated that a Au surface covered with a SAM of 3 exhibited no detectable change in surface wettability upon photoisomerization in the absence of MV 2+ CB[8] ( Supplementary Fig. S11 ), confirming that the light-switchable surface wettability was indeed caused from the reversible dissociation/reformation of the heteroternary complex. This reversible light-induced switch of fluorescence and non-fluorescence, as well as the oscillation in surface wettability ( Supplementary Fig. S12 ), could be repeated for at least three cycles without any obvious decay. In addition, the ‘on’ and ‘off’ photoswitching (1,1)↔(0,0) represents a writing-erasing mechanism required for data storage in a memory device. In parallel, the redox-controlled dissociation and reformation of (MV 2+ F· trans - 3 ) CB[8] on the surface was also investigated. Using the heteroternary complex terminated substrate as the working electrode with MV 2+ F CB[8] (0.1 mM) in a phosphate buffer (0.1 M pH=7) as the supporting electrolyte, the fluorescent pattern was completely removed when a potential (−0.7 V versus SCE) was applied ( Fig. 5b , (1,1)→(0,1)), and the hydrophobicity of the Au surface recovered ( θ =92°). It is believed that the homoternary complexation of (MV +· F) 2 CB[8] drives the fluorescent viologen derivative away from the trans - 3 -terminated substrate, resulting in a (0,1) state. In contrast to the cis - 3 -terminated substrate resulting from UV photoirradiation, the trans - 3 -terminated substrate is still capable of binding other first-guest CB[8] complexes, thus distinguishing the electrochemical switch (1,1)→(0,1) from the photochemical one (1,1)→(0,0). The subsequent reoxidation (applied potential: −0.3 V versus SCE) brought back both the fluorescent pattern and the hydrophilicity of the Au surface ( θ =68°) upon reformation of (MV 2+ F· trans - 3 ) CB[8] on a surface. This particular ‘on’ and ‘off’ electrochemical switching (1,1)↔(0,1) represents an orthogonal writing-erasing mechanism to that of the photo-switch and can be potentially employed simultaneously to greatly increase the complex structure (message) written on a surface. As both the photochemical and the electrochemical processes are fully reversible, the order of the external inputs only displays different outcomes but does not limit the direction of switching represented in Fig. 5a . Complementarily, we also formed the heteroternary complex on a surface by first immobilizing a viologen ligand ( 5 ) on the Au surface followed by a sequential addition of CB[8] and dye-labelled azobenzene second guest 4 ( Supplementary Fig. S13 ) [43] , [47] . The orthogonal switching of the heteroternary complex on the surface was confirmed by the disappearance and reappearance of linear fluorescent patterns, however, this approach sacrifices the modulation of surface wettability and hence serves as a complementary experiment. By incorporating both redox- and light-responsive components into a single addressable supramolecular entity, a CB[8]-mediated host–guest complex has been shown to respond orthogonally to distinctly different stimuli through light-driven isomerization and redox-driven dimerization. Fully controlled switches between a ‘closed’ (1:1:1) heteroternary complex, a ‘closed’ (2:1) homoternary complex and a dissociated ‘open’ state have been demonstrated, which have the potential to be exploited in logic functions. Moreover, by designing a patterned substrate, orthogonal stimuli were amplified to tune surface properties that were readily visualized. The single CB[8] heteroternary complex thus offers a versatile platform for the next generation of chemical and biological devices with higher complexity. Materials All starting materials were purchased from Sigma Aldrich and used as received unless stated otherwise. CB[8], MV 2+ , N-(10-mercaptodecyl)- N '-methyl-4,4'-bipyridinium chloride ( 5 ) were prepared as documented previously [47] . Synthesis of 1 A solution of KOH (25 g, 380 mmol) and p -nitrophenol (5 g, 36 mmol) in water (6 ml) was heated at 120 °C for 1 h and then at 195–200 °C for 2 h (ref. 48 ). The mixture was cooled to room temperature and dissolved in water. The dark-red solution was acidified to pH=3 with concentrated HCl, extracted with Et 2 O and dried over Na 2 SO 4 . The filtered residue was recrystallized from EtOH/water (4:1, v/v) to give yellow crystals of 1 (2.3 g, 59.6%). 1 H NMR (400 MHz, d 6 -DMSO): δ (ppm)=10.09 (s, 2H), 7.72–7.70 (d, 4H), 6.94–6.92 (d, 4H). 13 C NMR (126 MHz, d 6 -DMSO): δ (ppm)=160.8, 146.1, 125.0, 116.6. ESI-MS ( m/z ): calcd. for C 12 H 10 N 2 O 2 , [M+H] + , 215.23; found: 215.25. Synthesis of 2 A solution of 2-[2-(2-chloroethoxy) ethoxy]ethanol (1.855 g, 11.00 mmol) in EtOH (5 ml) was added to an EtOH solution (30 ml) of KOH (561 mg, 10.00 mmol) and 4-phenylazophenol (1.982 g, 10 mmol) along with a catalytic amount of KI [49] . The mixture was refluxed for 16 h, cooled to room temperature and neutralized. The filtered residue was dissolved in CHCl 3 , washed with water and dried over MgSO 4 . The filtered residue was purified by chromatography (EtOAc/hexane (1:4)) and recrystallized from MeOH to give 2 (1.652 g, 50.0%). 1 H NMR (500 MHz, d 6 -DMSO): δ (ppm)=7.90–7.88 (d, 2H, ar), 7.85–7.84 (d, 2H, ar), 7.59–7.56 (m, 2H, ar), 7.54–7.51 (m, 1H, ar), 7.16–7.14 (m, 2H, ar), 4.59–4.56 (d, 2H), 4.23–4.21 (d, 2H), 3.80–3.78 (d, 2H), 3.69–3.65 (d, 2H), 3.62–3.60 (d, 2H), 3.50–3.48 (d, 2H). 13 C NMR (126 MHz, d 6 -DMSO): δ (ppm)=161.3, 152.0, 146.2, 130.8, 129.4, 124.6, 122.3, 115.1, 70.5, 70.0, 69.8, 68.8, 67.7, 60.2. ESI-MS ( m/z ): calculated for C 18 H 22 N 2 O 4 , [M+H] + , 331.34; found: 331.39. Synthesis of 3 To a DMF solution (25 ml) of 4-(phenyldiazenyl)phenol (2.100 g, 10.59 mmol) and potassium t -butoxide (1.249 g, 11.13 mmol), 11-bromo-1-undecene (2.44 ml, 11.13 mmol) was added [50] . The mixture was refluxed for 10 min, cooled to room temperature, poured into water (100 ml) and extracted with hexane (4 × 50 ml). The organic phase was dried over Mg 2 SO 4 and the filtered residue was purified by chromatography (EtOAc:hexane, 1:20) to give 3a (2.389 g, 64.4%). A toluene (20 ml) solution of 3a (1 g, 2.85 mmol), AIBN (141 mg, 0.86 mmol) and thioacetic acid (873 mg, 11.47 mmol) was refluxed for 1 h, cooled to room temperature, poured into saturated NaHCO 3 (100 ml) and toluene (50 ml) solution. The organic phase was washed with water (4 × 5 ml) and dried over Mg 2 SO 4 . The filtered residue was purified by chromatography (EtOAc:hexane, 1:15) to give 3b (205 mg, 16.8%). A mixed MeOH (4 ml) and 1 M HCl in MeOH (1 ml) solution of 3b was refluxed for 5 h, cooled to room temperature and dried to give quantitative 3 . 1 H NMR (500 MHz, CDCl 3 ): δ (ppm)=7.92–7.90 (d, 2H), 7.88–7.87 (d, 2H), 7.51–7.48 (m, 2H), 7.45–7.42 (m, 1H), 7.01–6.99 (m, 2H), 4.05–4.03 (t, 2H), 2.88–2.85 (t, 2H), 2.32 (s, 3H, CH 3 ), 1.85–1.79 (m, 2H), 1.59–1.54 (m, 2H), 1.51–1.45 (m, 2H), 1.37–1.29 (m, 12H), 13 C NMR (126 MHz, CDCl 3 ): δ (ppm)=161.88, 152.92, 146.98, 130.44, 129.17, 124.91, 122.67, 114.85, 68.51, 30.80, 29.65, 29.62, 29.59, 29.50, 29.33, 29.30, 29.25, 28.96, 26.15. Synthesis of 4 A MeCN solution (100 ml) of 4-(phenyldiazenyl)phenol (2.10 g, 10.59 mmol), 2-bromoethanamine hydrochloride (1.90 g, 11.84 mmol), potassium carbonate (3.51 g, 25.40 mmol) along with a catalytic amount of 18-crown-6 was refluxed for 36 h, cooled to room temperature, and extracted into DCM (2 × 100 ml) and 1 M HCl (100 ml). The organic extracts were washed with water and brine, dried over MgSO 4 . The filtered residue was purified by chromatography (EtOAc/petroleum ether (40:60), 5:95) to a give 4a (1.56 g, 61%). 1 H NMR (400 MHz, CDCl 3 ): δ (ppm)=7.99–7.97 (d, 2H, ar), 7.86–7.84 (d, 2H, ar), 7.56–7.53 (m, 2H, ar), 7.51–7.49 (m, 1H, ar), 7.16–7.14 (m, 2H, ar), 4.27–4.24 (t, 2H, CH 2 ), 3.42–3.39 (t, 2H, CH 2 ). 13 C NMR (126 MHz, CDCl 3 ): δ (ppm)=161.1, 152.9, 144.6, 130.3, 129.2, 123.6, 123.4, 114.6, 71.3, 41.4. An aqueous solution (10 ml) of 4a (27.6 mg, 0.10 mmol) and FITC (390 mg, 1 mmol) was stirred at room temperature for 3 days. The crude product was purified on a Varian 940-LC with a linear gradient of 5–95 % B in 30 min with the maximum absorbance at 363 nm. The mobile phases were H 2 O (eluent A) and MeCN (eluent B), respectively. Synthesis of MV 2+ F N -methyl-4,4'-bipyridinium iodide [47] (2 g, 6.70 mmol) and 2-bromoethanamine hydrochloride (1.300 g, 8.10 mmol) were refluxed in MeCN for 3 days. The precipitant was filtered and washed with MeCN and dried under vacuum. 1 H NMR (400 MHz, d 7 -DMF): δ (ppm)=9.62–9.60 (d, 2H, ar), 9.55–9.53 (d, 2H, ar), 9.02–9.01 (d, 2H, ar), 8.97–8.96 (d, 2H, ar), 5.13–5.16 (t, 2H, CH 2 ), 4.72 (s, 3H, CH 3 ) 3.69–3.66 (t, 2H, CH 2 ). 13 C NMR (126 MHz, d 6 -DMSO): δ (ppm)=151.1, 150.9, 146.6, 146.3, 126.4, 126.3, 49.3, 48.1, 39.4. An aqueous solution (10 ml) of the resulting compound (45.8 mg, 0.10 mmol) and FITC (390 mg, 1 mmol) was stirred at room temperature for 3 days. KPF 6 (73.6 mg, 0.40 mmol) was added to the solution and the precipitate was filtered off and washed with water, dried under vacuum. The crude was dissolved in 5 ml acetone, a solution of n-Bu 4 NCl (11.1 mg, 0.40 mmol) in 2 ml acetone was then added, and the precipitate was filtered off and washed with water, dried under vacuum to give MV 2+ F (32.43 mg, 48%). 1 H NMR (d 7 -DMF): δ (ppm)=9.68–9.66 (d, 2H, viologen (v)), 9.56–9.52 (d, 2H, ar, v), 9.07–9.04 (d, 2H, ar, v), 8.99–8.96 (d, 2H, ar, v), 8.23–6.61 (9H, ar, Fluorescein), 5.25–5.22 (t, 2H, CH 2 ), 4.71 (s, 3H, CH 3 , v) 4.48–4.47 (t, 2H, CH 2 ). General preparation for surface experiments For unpatterned substrates, Au substrates were directly immersed into EtOH solutions of mixed thiols (decanethiol: 3 , 8:1) under nitrogen atmosphere for 18 h. For patterned substrates, PDMS stamps were wetted by EtOH solutions of decanethiol (2 mM) and then placed onto Au substrates for 30 s. After peeling away the stamps, the resulting substrates were washed by EtOH and immersed into solutions of mixed thiols (decanethiol: 3 , 8:1) in EtOH (2 mM) under nitrogen atmosphere for 5 min. The resulting substrates were washed by EtOH, immersed into an aqueous solution (0.25 mM) of MV 2+ /(MV 2+ F) CB[8], and left on a shaker with 200 r.p.m. for 5 min. The resulting substrates were washed by water and dried under nitrogen. For the complementary experiment, 5 was μCPed on a Au substrate after CB[8] was threaded on to a 4 -terminated Au substrate [47] . Instrumentation 1 H NMR (400 MHz) spectra and 1 H NMR (500 MHz), 13 C NMR, DOSY and HMQC spectra were recorded on a Bruker Avance QNP 400 and 500 MHz Ultrashield equipped with a 5-mm BBO ATM probe with a z-gradient, respectively. ESI-MS was performed on a Fischer Thermo Scientific LTQ Velos Ion Trap Mass Spectrometer. HPLC was performed on a Varian 940LC. UV–vis spectra were recorded on a Varian Cary 4000 UV–vis spectrophotometer. Fluorescence microscopy was performed on a Leica DMI 4000B microscope. Cyclic voltammetry was carried out on a PGSTAT30 Potentiostat (EcoChemie) with a GPES electrochemical interface. The working electrode was a glassy carbon disk (3 mm diameter) and the counter electrode was a platinum wire. Spectroelectrochemistry was performed by combining a Varian Cary 4000 spectrophotometer with a PGSTAT30 Potentiostat. An ITO glass electrode was used as the working electrode. Contact angle measurements were performed on a KSV CAM 200 goniometer. Photoirradiation was performed on a LZC-ORG photoreactor with both 350 and 420 nm wavelength lamps. Titration experiments were carried out on a ITC200 from Microcal Inc. How to cite this article: Tian, F. et al. Orthogonal switching of a single supramolecular complex. Nat. Commun. 3:1207 doi: 10.1038/ncomms2198 (2012).